A synthetic icosahedral DNA-based host–cargo complex for functionalin vivoimaging The encapsulation of molecular cargo within well-defined supramolecular architectures is highly challenging. Synthetic hosts are desirable because of their well-defined nature and addressability. Encapsulation of biomacromolecules within synthetic hosts is especially challenging because of the former's large size, sensitive nature, retention of functionality post-encapsulation and demonstration of control over the cargo. Here we encapsulate a fluorescent biopolymer that functions as a pH reporter within synthetic, DNA-based icosahedral host without molecular recognition between host and cargo. Only those cells bearing receptors for the DNA casing of the host–cargo complex engulf it. We show that the encapsulated cargo is therefore uptaken cell specifically in Caenorhabditis elegans . Retention of functionality of the encapsulated cargo is quantitatively demonstrated by spatially mapping pH changes associated with endosomal maturation within the coelomocytes of C. elegans . This is the first demonstration of functionality and emergent behaviour of a synthetic host–cargo complex in vivo . Synthetic host scaffolds present exciting possibilities for emergent behaviour [1] given their amenability to encapsulate functional guests. In host–guest complexes, two independent entities are supramolecularly associated resulting typically in the entrapment of one of these (guest or cargo) inside the available volume of the other (host) [2] . Host–guest complexes based on synthetic molecular hosts, such as cyclodextrins [3] , calixarenes [4] , cucurbiturils [5] , porphyrins [6] , crown ethers [7] , zeolites [8] and cryptands [9] , form structurally well-defined, synthetic scaffolds. A general strategy to achieve encapsulation within synthetic hosts involves the controlled polymerization of host units resulting in a well-defined cavity within which the guest (cargo) is accommodated and stabilized by molecular recognition [2] . Recently, bio-inspired peptide scaffolds, based on viral proteins that mimic naturally occurring hosts like viruses, have emerged as promising synthetic hosts [10] . Controlled oligomerization of DNA motifs into well-defined polyhedra enclosing well-defined cavities has been also recently demonstrated [11] , [12] , [13] , [14] , [15] , [16] , [17] , [18] , [19] , [20] . However, the potential of DNA polyhedra as synthetic molecular hosts for encapsulating functional cargo has remained unexplored, despite the internal cavity being utilizable [21] , [22] , [23] . Our previous studies had established that DNA motifs comprising five-way junctions could undergo oligomerization resulting in a well-defined DNA icosahedron [22] . The advantage of a synthetic host based on a biological material such as DNA is that they may be used to construct host–cargo complexes whose functionality may be demonstrated in living systems. Further, a molecular recognition-free route to achieve this would enable a strategy that is generalizable to many types of functional cargo. Importantly, the functionality of the cargo post-encapsulation should be quantitatively demonstrable in vivo . We therefore chose Fluorescein isothiocyanate (FITC)-Dextran (FD) as a cargo as it satisfied the aforementioned criteria, as it possesses the following two properties. First, the fluorescein moieties (FITC) on FD are pH sensitive, conferring on it the property to measure organellar pH inside living cells and whole organisms [24] , [25] . Second, this neutral biopolymer does not interact with membrane-bound receptors and this confers on it the property to mark the fluid phase endocytic pathway [26] . Importantly, non-functionalized FD cannot be targeted to specific endocytic pathways because of this non-interacting property. Thus, any emergent properties of the cargo (FD) on encapsulation in DNA polyhedra may be measurable in terms of altered endocytic properties of the resultant DNA host–cargo complex. Simultaneously, cargo functionality post-encapsulation within a living system may be quantitatively evaluated in terms of the other property, that is, pH mapping ability. We thus proceeded to study: whether 10-kDa FITC-Dextran (FD10) could be encapsulated inside a synthetic, icosahedral DNA host; whether the resultant host–cargo complex showed any emergent behaviour reflected in entirely new endocytic routes of uptake for FD10; and whether the functionality of the cargo in terms of pH sensing properties is preserved along with any manifested emergent property within a living organism. Here we report the formation of a synthetic icosahedral DNA host–cargo complex and demonstrate the retention of the functionality of the encapsulated cargo along with emergent behaviour within a living organism. We probed the nature of association of the encapsulated cargo with the host scaffold within the host–cargo complex and find that the cargo shows minimal interaction with the host scaffold. Emergent properties of the host–cargo complex in cellulo were manifested in dramatic alteration of uptake pathways of encapsulated FD10 versus free FD10 in Drosophila hemocytes. Free FD10 is uptaken by the fluid phase pathway, whereas encapsulated FD10 was uptaken exclusively by the anionic ligand-binding receptor (ALBR) pathway indicating that encapsulated FD10 was now targeted to ALBRs. This was also borne out in vivo , where the host–cargo complex was uptaken only by specific cells (coelomocytes) in Caenorhabditis elegans that expressed ALBRs. The functionality of the encapsulated cargo in vivo was quantitatively demonstrated by mapping pH changes associated with endosomal maturation [27] along the ALBR pathway in coelomocytes of C. elegans . Complex formation between DNA icosahedron and FD10 DNA icosahedra were assembled using the reported modular assembly protocol, which involves the association of two types of five-way junctions V and U (or V and L) to first form half icosahedra VU 5 (or VL 5 ) followed by the further assembly of 1:1 VU 5 :VL 5 ( Fig. 1a ; Supplementary Fig. S1 ) into icosahedral DNA nanocapsules, I, in near quantitative yields [22] . To encapsulate the cargo, FD10, inside these icosahedral capsules, the two halves VU 5 and VL 5 were incubated in 1:1 ratio in presence of 2 mM FD10, such that there is at least one FD10 molecule per 1,000 nm 3 , which is the measured minimum encapsulable volume of the DNA icosahedron ( Fig. 1a ) [22] . On ligation, the excess free FD10 was separated from DNA icosahedra by gel electrophoresis followed by size-exclusion chromatography (SEC)–high-performance liquid chromatography (HPLC; Fig. 1b ). This yielded DNA icosahedra that showed fluorescence corresponding to FD10, despite rigorous purification from free FD10, suggesting the formation of an I FD10 complex. The ratio of absorbance at 254–488 nm of the eluted fraction corresponding to the I FD10 complex gave a stoichiometry of FD10:I of 2:1 indicating an average of two FD10 molecules associated per DNA cage ( Fig. 1b,d ). 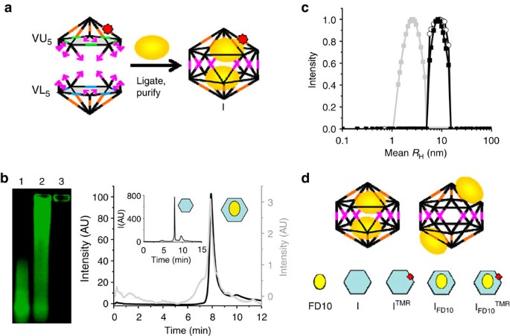Figure 1: Formation and characterization of host–cargo complex of DNA icosahedron and FD10. (a) Schematic illustration of the formation of FD10-loaded icosahedra (IFD10). Two complementary half icosahedra VU5and VL5are mixed in a 1:1 ratio in 2 mM FD10 solution and purified from free FD10. (b) (Left) Gel electrophoretic mobility shift assay for the formation of IFD10. 0.8% agarose gel (1× TAE) showing association of FD10 with icosahedron: lane 1, FD10; lane 2, 1:1 (VU5: VL5)+2 mM FD10 post ligation; lane 3, purified IFD10. Gel was visualized using FITC excitation. (Right) Size-exclusion chromatogram (SEC-HPLC) of IFD10complex post-gel excision. SEC traces were followed at 254 nm (black) and 488 nm (grey). Inset: SEC of standard, reference sample of unlabelled, unloaded icosahedron I (retention time 8 min). (c) DLS traces of free FD10 (grey squares), the standard sample of DNA icosahedra, I (open black circles) and purified IFD10complex (black squares). (d) Possible modes of association of cargo (FD10) with the host DNA capsule. Also given are cartoons representing all the species used in the present study. Figure 1: Formation and characterization of host–cargo complex of DNA icosahedron and FD10. ( a ) Schematic illustration of the formation of FD10-loaded icosahedra (I FD10 ). Two complementary half icosahedra VU 5 and VL 5 are mixed in a 1:1 ratio in 2 mM FD10 solution and purified from free FD10. ( b ) (Left) Gel electrophoretic mobility shift assay for the formation of I FD10 . 0.8% agarose gel (1× TAE) showing association of FD10 with icosahedron: lane 1, FD10; lane 2, 1:1 (VU 5 : VL 5 )+2 mM FD10 post ligation; lane 3, purified I FD10 . Gel was visualized using FITC excitation. (Right) Size-exclusion chromatogram (SEC-HPLC) of I FD10 complex post-gel excision. SEC traces were followed at 254 nm (black) and 488 nm (grey). Inset: SEC of standard, reference sample of unlabelled, unloaded icosahedron I (retention time 8 min). ( c ) DLS traces of free FD10 (grey squares), the standard sample of DNA icosahedra, I (open black circles) and purified I FD10 complex (black squares). ( d ) Possible modes of association of cargo (FD10) with the host DNA capsule. Also given are cartoons representing all the species used in the present study. Full size image To determine the nature of association of FD10 with the DNA icosahedron, I, the I FD10 complex was characterized by dynamic light scattering (DLS). DLS of a sample of pure FD10 showed peaks corresponding to an R H of 2.6±1.0 nm ( Fig. 1c ). DLS of a sample of DNA icosahedra, I, showed an R H of 9.2±0.1 nm. DLS of a pure sample of I FD10 complex showed an R H of 9.3±0.4 nm, consistent with the measured dimensions of the DNA icosahedron [22] . There were no peaks at R H ~3 nm corresponding to free FD10 ( Fig. 1c ). FD10 is encapsulated within DNA icosahedra The I FD10 complex could have the FD10 externally associated or internally entrapped within the DNA Icosahedron ( Fig. 1d ). The former would show an altered hydrodynamic radius by DLS, which is not observed. To confirm the latter model, we subjected the I FD10 complex (I FD10 ) to quenchers of different sizes ranging from 0.5 to 5 nm diameter and studied their abilities to quench the fluorescence of the fluorescein moiety by collisional quenching. In the absence of any added quencher, fluorescence lifetime of DNA-associated FD10 (I FD10 ) was the same as free FD10 (inset, Fig. 2b ), indicating that the fluorophore in I FD10 is unaffected by the DNA scaffold I ( Supplementary Fig. S2 ). Next, the fluorescence intensity was monitored by the addition of quenchers of different sizes to a solution of I FD10 . If the FD10 is encapsulated within the DNA icosahedra, only quenchers smaller than the measured pore size will be able to access the interior of the polyhedron and quench the fluorescence, whereas quenchers larger than the pore size will not. I FD10 and FD10 (50 nM each) were treated with quenchers of various sizes, such as iodide (0.35 nm), amino TEMPO (1 nm), Nanogold (1.5 nm) and gold nanoparticles of sizes 2, 3, 4 and 5 nm, respectively. Each species of quencher has an intrinsically different ability to collisionally quench fluorescence and this was corrected for by using that concentration of the quencher, which results in a 50% decrease in fluorescence intensity of the sample. This was obtained from the reciprocal of their measured Stern-Volmer constants ( K SV , Supplementary Table S1 and Supplementary Fig. S3 ) [28] . When FD10 and I FD10 (50 nM each) were subjected to 1/ K SV concentration of each quencher, it was observed that in the case of FD10, quenchers of all sizes quenched the fluorescence intensity by 50% ( Fig. 2a ). However, in the case of I FD10 , only quenchers below ~2.2 nm diameter could quench the fluorescence by 50%. Quenchers of sizes ≥ 3 nm were ineffective at quenching fluorescence, whereas quenchers between 2.2 and 3 nm diameters could only partially quench fluorescence ( Fig. 2a ). This was further confirmed by an analogous study of fluorescence lifetimes of the fluorescein moieties present on free FD10 and I FD10 ( Fig. 2b ). Fluorophore lifetime is a direct reporter of the quenching environment of the fluorophore and the mechanism of fluorescence quenching by different quenchers [29] . Fluorescein lifetime in I FD10 and free FD10 showed comparable decrease for small sized quenchers, whereas quenchers larger than 3 nm diameter could not decrease the lifetime for I FD10 ( Fig. 2b ). 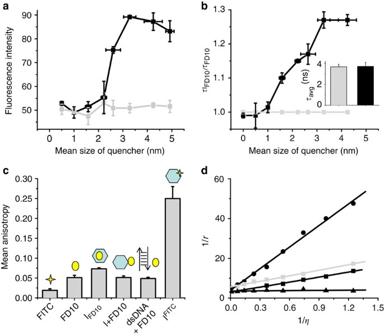Figure 2: Accessibility of FD10 in the host–cargo complex and interaction of encapsulated cargo within the host capsule. (a) Fluorescence intensity-based quenching assay for free FD10 (grey squares) and IFD10complex (black squares). All quenchers are gold nanoparticles (GNPs) of indicated sizes except iodide (0.5 nm), TEMPO-A (1 nm) and TEMPO-Dextran (2.5 nm). Mean values of two experiments are presented, with their corresponding s.d. (b) Fluorescence lifetime measurements of free FD10 (grey squares) and IFD10complex (black squares) with the same quenchers. Mean values of two independent experiments are presented, along with their s.d. Inset: the lifetimes of free (grey bar) and encapsulated (black bar) FD10 in absence of any quencher. Error bars indicate s.d. (c) Fluorescence anisotropy of free FITC, FD10, IFD10, externally added FD10 to preformed I and double-strand DNA (dsDNA), and IFITC. Each bar represents mean of three independent experiments, with their associated s.d. (d) Perrin plot showing rotational correlation times of FITC (black circles), FD10 (grey squares), IFD10(black squares) and IFITC(black triangles). Figure 2: Accessibility of FD10 in the host–cargo complex and interaction of encapsulated cargo within the host capsule. ( a ) Fluorescence intensity-based quenching assay for free FD10 (grey squares) and I FD10 complex (black squares). All quenchers are gold nanoparticles (GNPs) of indicated sizes except iodide (0.5 nm), TEMPO-A (1 nm) and TEMPO-Dextran (2.5 nm). Mean values of two experiments are presented, with their corresponding s.d. ( b ) Fluorescence lifetime measurements of free FD10 (grey squares) and I FD10 complex (black squares) with the same quenchers. Mean values of two independent experiments are presented, along with their s.d. Inset: the lifetimes of free (grey bar) and encapsulated (black bar) FD10 in absence of any quencher. Error bars indicate s.d. ( c ) Fluorescence anisotropy of free FITC, FD10, I FD10 , externally added FD10 to preformed I and double-strand DNA (dsDNA), and I FITC . Each bar represents mean of three independent experiments, with their associated s.d. ( d ) Perrin plot showing rotational correlation times of FITC (black circles), FD10 (grey squares), I FD10 (black squares) and I FITC (black triangles). Full size image Mobility of entrapped cargo within I FD10 To further probe the nature of association of the FD10 cargo with its synthetic host I, fluorescence anisotropy of fluorescein moieties present on entrapped FD10 was monitored. This reports on segmental motion as well as global rotation corresponding to dextran tumbling. Both rotations cause fluorescence depolarization, which is reflected in fluorescence anisotropy [30] . As shown in Figure 2c , the fluorescein moieties of FD10 showed an anisotropy of 0.05±0.01, which suggest that in FD10, the major component of the anisotropy of fluorescein comes from the free segmental rotation as reflected in the low anisotropy values ( Supplementary Fig. S4 ). Interestingly, in the I FD10 complex, fluorescein anisotropy was only marginally higher, 0.073±0.002, indicating that its motion is not affected on complexation with the DNA icosahedron. A 2:1 mixture of externally added FD10 to preform I showed anisotropy consistent with free FD10. This is further confirmed by anisotropy of a mixture of FD10 and linear, duplex DNA in the stoichiometry of the host –cargo complex, I FD10 . To check the extent of anisotropy increase when a fluorophore is actually attached to the DNA host, we compared anisotropies between I carrying a single FITC (I FITC ) and the I FD10 complex. The latter showed anisotropy of 0.073±0.003. I FITC was made by incorporating a FITC tag on one of the component oligonucleotides V 1 FITC of the 5WJ 'V' of the half icosahedron VU 5 . The anisotropy values of the fluorophore reflect its rotation while attached to the DNA structure, as it changes from V 1 FITC to I/2 FITC to I FITC ( Fig. 2c ; Supplementary Fig. S4 ). Thus, I FITC showed a much higher anisotropy of 0.25±0.03. To further explore the association of FD10 with I in the host–cargo complex, I FD10 , rotational correlation times ( θ ) of fluorescein present on free FD10 and I FD10 were determined. These are obtained by measuring anisotropy ( r ) of a sample as a function of viscosity ( η ) of the medium [30] . Samples were made in solutions containing well-defined proportions of glycerol in water that yielded solutions of defined viscosities, with a final fluorophore concentration of 50 nM. Anisotropies of these samples were plotted as a function of solution viscosity giving the Perrin plot for FITC, free FD10 and I FD10 , the slope of which gives the rotational correlation time ( θ ) of fluorescein in these samples ( Fig. 2d ). Free FD10 showed θ =2.2 ns, whereas that of I FD10 was θ =3.1 ns. Fluorescein covalently attached to the synthetic host in I FITC showed θ =140 ns. I FD10 is targeted to anionic ligand-binding receptors To see if encapsulation of FD10 within a host–cargo complex manifests different properties from free FD10, we proceeded to explore uptake properties of free and host-encapsulated FD10 in cellulo . Drosophila hemocytes are a widely used model system to study the mechanisms of endocytosis of different types of molecules ( Fig. 3a ) [26] . When Drosophila hemocytes were pulsed with 12 μM free FD10, the latter was found to be localized in punctate structures. This uptake in cells was quantified in terms of whole-cell intensity ( Fig. 3b ), as previously described [31] (see Methods). Hemocytes were then pulsed with 12 μM I FD10 (DNA: 3 μM, FD10: 12 μM) for 5 min and chased for 5 min. Fluorescence images of these cells ( Fig. 3c ) showed that I FD10 was similarly localized in punctate structures, which showed slightly higher uptake than free FD10. When hemocytes were pulsed with 12 μM free FD10 in the presence of excess maleylated BSA (mBSA), its uptake by hemocytes is unaffected as expected for fluid phase endocytosis, and consistent with previous studies [26] . Interestingly, when hemocytes were pulsed similarly with 12 μM I FD10 (DNA: 3 μM, FD10: 12 μM) and excess mBSA, uptake is completely abolished and intensities are commensurate with the level of autofluorescence in the cells ( Fig. 3b ). When Drosophila hemocytes were pulsed with a sample of TMR-labelled DNA icosahedra loaded with FD10 (I FD10 TMR ), chased and imaged, they showed co-localization ( Fig. 3d ) of the synthetic DNA host (in the TMR channel) and cargo FD10 (in the FITC channel). This confirms that when pulsed with I FD10 , the FD10 present in endosomes along this altered pathway is present along with its synthetic DNA host. 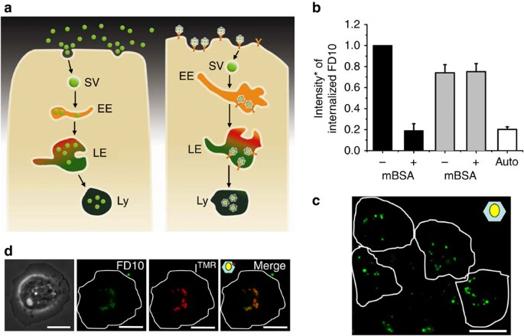Figure 3: Encapsulated FD10 is uptaken by anionic ligand-binding receptorsin cellulo.(a) Schematic showing the different pathways of endocytosis adopted by free and encapsulated FD10. EE, early endosome; LE, late endosome; Ly, lysosome; SV, spherical vesicle. (b) IFD10is endocytosed via the anionic ligand-binding receptor (ALBR) pathway in hemocytes. Cells were pulsed with FD10 and IFD10in the presence and absence of maleylated BSA (mBSA, 30 μM). Internalization was quantified in terms of mean fluorescence intensity of cells, normalized to the mean intensity of IFD10. The contribution from autofluorescence is also shown. Error bars indicate s.e.m. (n=25 cells). (c) Epifluorescence images showing internalization of IFD10inDrosophilahemocytes. Cells that are pulsed with IFD10for 5 min chased for 5 min and imaged, show distinct punctate structures containing IFD10. Scale bar, 10 μm. (d) FD10 is internalized in hemocytes while it is present inside the DNA cage. Cells, pulsed with IFD10TMR, chased for 5 min and imaged in the FITC channel (488 nm excitation, green) and TMR channel (554 nm excitation, red), show co-localization. Scale bar, 10 μm. *refers to normalized whole cell intensity. Figure 3: Encapsulated FD10 is uptaken by anionic ligand-binding receptors in cellulo. ( a ) Schematic showing the different pathways of endocytosis adopted by free and encapsulated FD10. EE, early endosome; LE, late endosome; Ly, lysosome; SV, spherical vesicle. ( b ) I FD10 is endocytosed via the anionic ligand-binding receptor (ALBR) pathway in hemocytes. Cells were pulsed with FD10 and I FD10 in the presence and absence of maleylated BSA (mBSA, 30 μM). Internalization was quantified in terms of mean fluorescence intensity of cells, normalized to the mean intensity of I FD10 . The contribution from autofluorescence is also shown. Error bars indicate s.e.m. ( n =25 cells). ( c ) Epifluorescence images showing internalization of I FD10 in Drosophila hemocytes. Cells that are pulsed with I FD10 for 5 min chased for 5 min and imaged, show distinct punctate structures containing I FD10 . Scale bar, 10 μm. ( d ) FD10 is internalized in hemocytes while it is present inside the DNA cage. Cells, pulsed with I FD10 TMR , chased for 5 min and imaged in the FITC channel (488 nm excitation, green) and TMR channel (554 nm excitation, red), show co-localization. Scale bar, 10 μm. *refers to normalized whole cell intensity. Full size image Altered endocytic uptake of I FD10 is manifested in vivo Given the stark alteration of molecular interactions and hence endocytic uptake pathways between free and encapsulated cargo in cellulo , we proceeded to see whether this was also observed in vivo . We assessed the uptake of free FD10 and I FD10 inside C. elegans . C. elegans is a nematode that contains scavenger cells, called coelomocytes, which endocytose fluid from the pseudocoelom ( Supplementary Figs S5 and S6 ) [32] . When 15 μM free FD10 is microinjected into C. elegans , it is clear that there is highly nonspecific distribution of FD10 throughout the pseudocoelom ( Fig. 4a , upper panel). Injection of the same concentration of FD10 encapsulated in the host–cargo complex I FD10 (DNA: 3 μm, FD10: 15 μM), in complete contrast, shows specific uptake only by the coelomocytes ( Fig. 4a , lower panel and Supplementary Fig. S7 ). This was completely abolished when I FD10 was coinjected with mBSA ( Supplementary Figs S7 and S8 ). 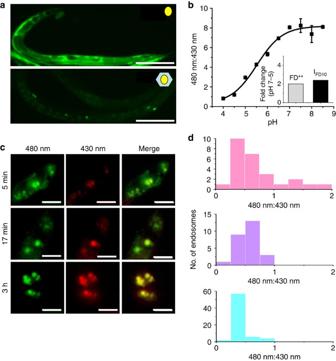Figure 4: Encapsulated FD10 uptaken by coelomocytes ofC. elegansis functional. (a) Representative image showing a wild type hermaphrodite microinjected with a solution of FD10 (upper panel) and IFD10(lower panel) into the pseudocoelom, from which it is uptaken by coelomocytes. Scale bar, 10 μm. (b)In vitropH calibration curve of IFD10obtained by dual excitation of fluorescein at 480 and 430 nm. Error bars indicate s.e.m of three measurements (n=10). Inset: fold change of FD and IFD10from pH 5 to 7in vivo.(c) Representative pseudocolour merged images of IFD10-labelled coelomocytes in wild type hermaphrodites at indicated times. Scale bar, 10 μm. (d) Histograms of 480:430 ratios of maturing endosomes, at 5 min (pink), 17 min (purple) and 3 h (cyan;n=25 endosomes; **Thein vivo foldchange for FD was obtained using FD70, as the uptake characteristics of FD10 was so poor thatin vivopH measurements were not possible to make with FD10). Figure 4: Encapsulated FD10 uptaken by coelomocytes of C. elegans is functional. ( a ) Representative image showing a wild type hermaphrodite microinjected with a solution of FD10 (upper panel) and I FD10 (lower panel) into the pseudocoelom, from which it is uptaken by coelomocytes. Scale bar, 10 μm. ( b ) In vitro pH calibration curve of I FD10 obtained by dual excitation of fluorescein at 480 and 430 nm. Error bars indicate s.e.m of three measurements ( n =10). Inset: fold change of FD and I FD10 from pH 5 to 7 in vivo. ( c ) Representative pseudocolour merged images of I FD10 -labelled coelomocytes in wild type hermaphrodites at indicated times. Scale bar, 10 μm. ( d ) Histograms of 480:430 ratios of maturing endosomes, at 5 min (pink), 17 min (purple) and 3 h (cyan; n =25 endosomes; **The in vivo fold change for FD was obtained using FD70, as the uptake characteristics of FD10 was so poor that in vivo pH measurements were not possible to make with FD10). Full size image Functionality of the cargo of I FD10 in vivo To confirm that the cargo (FD10) is still functional post-encapsulation within the DNA host and post-delivery in vivo , we measured the pH of I FD10 -containing compartments inside the coelomocytes. Fluorescein is a well-known fluorescent reporter of pH and intracellular pH measurements use dual excitation of fluorescein at 480 and 430 nm [24] . First, the in vitro pH calibration curve for I FD10 was generated for pH ranging from 4 to 8 ( Fig. 4b ). Further, the I FD10 complex was microinjected in worms and these worms were immersed in pH clamping buffers containing the ionophore nigericin at pH 7 and 5 for 75 min. This clamps the pH of the endosomes in coelomocytes to the pH of the external buffer ( Supplementary Fig. S9a ). The coelomocytes were imaged using dual excitation method [24] . The fold change in 480:430 emission ratio of both free and encapsulated FD10 remains unaltered in vivo (inset, Fig. 4b ). Also, the fold change in 480:430 emission ratio for I FD10 remains unchanged in vitro , as well as in vivo ( Supplementary Fig. S9b ). Cumulatively, these indicate that the functionality of FD10 post-encapsulation is quantitatively preserved. The functionality of the encapsulated FD10 in living worms under native conditions was demonstrated by the ability of I FD10 to map pH changes during endosomal maturation along the ALBR pathway in coelomocytes. The 480:430 ratio of ~35 endosomes in coelomocytes that were marked by I FD10 at 5, 17 min and 3 h post injection ( Fig. 4c ) gave a distribution as shown in Figure 4d . The in vivo pH of compartments containing I FD10 at 3 h post injection gave a 480:430 ratio of 2.5 that corresponded to a pH of ~5.2. This is consistent with I FD10 residing predominantly in the lysosomes, at 3 h, that are shown to have pH ~5.0 (ref. 27 ). We have demonstrated the encapsulation of a functional biomolecular cargo within a synthetic DNA host capsule of well-defined structure. Encapsulation to form a synthetic host–cargo complex is a molecular recognition-free strategy, which is generalizable to many types of functional cargo. Encapsulation relies mainly on size compatibility between the host and cargo ( Supplementary Table S2 ). The encapsulation studies indicate that for a cargo such as FD10, of size 5.2 nm, the presence of excess FD10 does not impede the formation of DNA icosahedra in solution and the FD10 molecules are associated with the capsules in a manner that does not significantly alter the size of the icosahedral DNA capsule. Post-encapsulation, quenching studies reveal that the FD10 present within the DNA cage is inaccessible to particles >3 nm in size, completely accessible to particles below 2 nm, whereas particles between 2 and 3 nm have limited access. Such size-dependent quenching has been observed in the case of the fluorophores present inside the endoplasmic reticulum where the transition point corresponds to the average pore size of the translocon, the protein conduction channel present on the endoplasmic reticulum [33] . Given that the pore size of I has been shown to be ~2.5 nm experimentally and 2.8 nm by a theoretical model [22] , these studies confirm that FD10 is encapsulated as cargo within the DNA icosahedron as a host in the I FD10 complex. Anisotropy studies to probe the mobility of the encapsulated cargo within the DNA host showed only a very minor increase in anisotropy between free and encapsulated FD10. Such a meagre increase could also arise from weak interactions between FD10 and I that could be captured by measuring the probe lifetime of the cargo because of the quenching ability of the DNA host. However, free FD10 and I FD10 showed similar fluorescence lifetimes within experimental error (inset, Fig. 2b ), confirming that anisotropy clearly reports on the motion of the probe. This reveals that any potential weak interactions between FD10 and DNA scaffolds are not responsible for the mild increase in anisotropy seen in the host–cargo complex. These were complemented by studies on the rotational correlation times between free and encapsulated cargo. Here too, only a very small change in rotational correlation time ( θ ) of ~1 ns between free and encapsulated FD10 is observed, revealing that the entrapped FD10 molecule is very weakly associated with the synthetic icosahedral DNA host, I. Cumulatively, the studies on anisotropy and rotational correlation times suggest a model where the FD10 encapsulated inside the central void experiences only slightly hindered rotation due to its confined environment ( Fig. 2c,d ) . In Drosophila hemocytes and many other cell types, free FD10 does not engage any membrane receptor and is therefore endocytosed only along with the external bulk solution, thus marking the fluid phase ( Fig. 3a ) [26] . mBSA is a polyanionic molecule that is endocytosed exclusively by the ALBR pathway and thus does not compete out the uptake of free FD10 due to their uptake by completely independent pathways [26] . Our previous studies have established that DNA nanostructures are endocytosed via the ALBR pathway in Drosophila hemocytes, and are efficiently competed out by mBSA [31] . Our studies on the endocytic uptake of encapsulated FD10 in Drosophila hemocytes revealed that it was uptaken exclusively by the ALBR pathway, showing a dramatic change in uptake properties from free FD10 that is internalized by the fluid phase pathway. It is notable that without any chemical modification per se to the cargo, and mere physical encapsulation within a synthetic DNA host, an entirely new set of biochemical interactions is made available to the cargo resulting in a complete alteration of its natural endocytic property. The amplification of such a small difference in chemical terms to the cargo into an incommensurable difference in the host–cargo complex in terms of biochemical interactions in the context of a more complex system is the hallmark of emergent behaviour. This altered endocytic behaviour shown by the DNA host–cargo complex was also borne out in vivo . Coelomocytes of C. elegans express anionic ligand-binding receptors that internalize negatively charged entities such as DNA nanostructures by receptor-mediated endocytosis [34] . Competition experiments of I FD10 uptake in coelomocytes of C. elegans involving coinjection of I FD10 with excess of mBSA clearly revealed that it was uptaken via the ALBR pathway as against fluid phase endocytosis for free FD10 ( Supplementary Fig. S8 ). Here again the DNA host–cargo complex shows a key signature of emergent behaviour, that in the context of a more complex system, new properties emerge that could not be predicted in a simpler system. Thus, not only is the altered endocytic pathway manifested in vivo , but also targeting the cargo to only those cells of the organism that possess the relevant receptor is observed. This targeting behaviour and hence uptake of I FD10 is abolished when coinjected with mBSA that competitively binds to the relevant receptors ( Supplementary Fig. S8 ), demonstrating control over the cargo by manipulation of the synthetic host–organism interactions. Cargo functionality post-encapsulation and post-delivery into endosomes on the ALBR pathway in coelomocytes of C. elegans was checked by assessing its ability to map spatiotemporal pH changes associated with maturation of the endosomes that it marks. pH clamping of coelomocytes labelled with I FD10 at pH 5 and 7 showed that the in vivo fold change in 480:430 emission of the cargo was unchanged from the in vitro values. A time-dependent study on endosomal pH values showed characteristic, progressively narrowing pH distributions accompanied by acidification as the endosomes matured from the early endosomes to late endosomes to the lysosome, where the pH is tightly regulated. FD10 has two properties, one of non-targeted endocytic uptake by the fluid phase and another of pH sensitivity. It is important to note that emergent behaviour is observed in the case of the former but not in the latter. To our knowledge, this is the first in vivo observation of predicted emergent behaviour that has been the driving force for the construction of synthetic host–cargo systems [1] . The exquisite engineerability of a DNA-based synthetic host scaffold [23] , [35] makes this class of host–cargo complexes amenable to invoking different host–organism interactions. Thus, combinatorial possibilities to generate different host–cargo complexes based on DNA polyhedra could yield several types of emergent properties that are controllable. Such controllable emergent behaviour of host–cargo complexes would position the latter as powerful probes or tools to interrogate biological phenomena both in living cells and whole organisms. Materials Labelled and unlabelled oligonucleotides were obtained from IBA-GmBh and Bioserve, respectively. FITC dextrans, TD155 and nigericin were purchased from Sigma; TD10 was obtained from Invitrogen. mBSA and N -cyano imidazole were synthesized in-house according to previous protocols [26] , [36] . Methods for DNA icosahedron construction and characterization have been previously described [22] . Encapsulation of molecular cargo within DNA icosahedron The two half icosahedra VU 5 and VL 5 (3.33 μM each) were mixed in presence of 2 mM of the desired cargo, that is, FD (FD4, 10, 20, 40, 70 and 150) in 10 mM phosphate buffer, pH 6, incubated at 45 °C for 4 h and annealed to room temperature. After incubation for 72 h at 4 °C, it was chemically ligated using N -cyano imidazole [36] at room temperature and again incubated for 72 h at 4 °C. Thereafter, the solution containing DNA host (I) and cargo (FD10) was run on 0.8% agarose gel in 1X TAE buffer. The band corresponding to I was excised and eluted in 100 mM NaCl and 1 mM MgCl 2 . The eluted solution was further purified by either size-exclusion chromatography [22] (BioSep S3000, Phenomenex) on a Shimadzu HPLC system (Shimadzu) or dialysis using a 50-kDa MWCO CelluSep membrane (MFPI) to remove trace amounts of free cargo (FD10) from the DNA host–cargo complex (I FD10 ). DLS experiments DLS studies were performed on a DynaPro-99 unit (Protein Solutions) at 25 °C. Buffers and samples (FD10, I FD10 , I) were filtered using 0.02 μm filters (Whatman) and 0.22 μM filters (Millipore), respectively and spun at 10,000 r.p.m. for 10 min before use. The experimental settings used were: acquisition time, 3 s; S/N threshold, 2.5; and sensitivity, 70%. The sample was illuminated with an 829.4 nm laser; scattering intensity at 90° and its autocorrelation function were measured simultaneously. Fluctuations >15% in the scattering intensity were excluded from the analysis. The DynaLS software (Protein Solutions) was used to resolve acquisitions into well-defined Gaussian distributions of hydrodynamic radii. The size of FD10 was measured at 1 mM concentration, whereas those of I FD10 and I were measured at 1 μM concentration of host. Anisotropy and Perrin plot measurements Anisotropy experiments were performed using 50 nM of fluorophore per sample, on Fluorolog 3L instrument (Horiba Jobin Yvon), in which the polarizing angles are fixed (90°). Before each experiment, the g factor was calibrated using FITC as a standard. For every sample, time series of anisotropy was acquired, and the mean of each time series was selected. For Perrin plot, the samples were prepared in 0, 10, 20, 30, 40, 50, 60, 70, 80 and 90% glycerol (w/v), maintaining the fluorophore concentration at 50 nM. Lifetime measurements Lifetime measurements were performed at 5 μM fluorophore concentration using a frequency domain Fluorolog Tau 3 (Horiba Jobin Yvon). The S and T channels were calibrated using glycogen as a standard and the operating frequency was 10 MHz. For each sample, the frequency and modulation spanned from 10 to 150 MHz using 7–10 intermediate frequency readings. The data obtained were fitted using the associated software and readings showing χ 2 value <1.2 were selected. Quencher characterization Quenchers of different sizes were selected based on literature reports; these included iodide (0.5 nm), amino TEMPO (1 nm) and nanogold (1.5 nm). Quenchers in the regime 2–5 nm are all gold nanoparticles and were synthesized using previously reported methods and characterized by transmission electron microscope [22] . The quencher of size ~2.5 nm was 1 kDa dextran (size=2.4–2.6 nm dia by DLS) that was coupled to carboxy TEMPO using dicyclohexylcarbodiimide and purified by SEC-HPLC. Fluorescence intensity and lifetime measurements For intensity-based quenching, the fluorescein concentration in FD10 and I FD10 was maintained at 50 nM in phosphate buffer of pH 7. All the quenchers were characterized from their measured Stern–Volmer plots for FD10. These concentrations of quenchers were added to FD10 and I FD10 . After addition of quencher, the solution was equilibrated for 2 min and fluorescence intensities measured. The percentage of fluorescence remaining was measured and plotted as percentage fluorescence. All readings were corrected for dilution. For lifetime measurements, the concentration of fluorescein in FD10 and I FD10 was maintained at 5 μM and quencher concentrations were increased accordingly. The lifetimes presented are average lifetimes in nanoseconds calculated from two component fitting of lifetimes using the formula: < τ avg >=( τ 1 f 1 2 + τ 2 f 2 2 )/( τ 1 f 1 + τ 2 f 2 ); where τ 1 and τ 2 are the lifetimes of two components and f 1 and f 2 are the respective fractions of the component [30] . Cell culture and in cellulo endocytic assays Drosophila hemocytes were isolated in complete medium using previously described methods [31] . Before pulsing, the cells were washed using Medium 1 (M1, 150 mM NaCl, 5 mM KCl, 1 mM CaCl 2 , 1 mM MgCl 2 , 20 mM HEPES, pH 7.0, supplemented with 1 mg ml −1 BSA and 2 mg ml −1 glucose). For pulsing, FD10 (12 μM), I FD10 (DNA: 3 μM, FD10:12 μM) or I FD10 TMR (DNA: 3 μM, FD10: 12 μM) in M1 buffer was added to these cells and incubated for 5 min. Labelling solution is then removed and replaced with M1 buffer for 5 min. After this, the cells are washed with M1 buffer and immediately imaged. Healthy cells were identified by the presence of well-developed lamellipodia. The area of lamellipodia was used to demarcate the perimeter of cells and drawn as a white line in fluorescent images indicating the perimeters of respective cells. For competition assays, hemocytes were divided into five plates. In the first plate, cells were untreated and used to measure autofluorescence. In two plates, cells were pulsed with FD10 and I FD10 . In the remaining two plates, the surface receptors were saturated with 30 μM mBSA for 5 min. After this, the cells were pulsed with I FD10 /FD10 (DNA: 3 μM, FD10: 12 μM), containing 30 μM mBSA for 5 min, chased, washed and imaged. Experiments were performed in duplicate. C. elegans strains and in vivo endocytic assays Standard methods were used to maintain C. elegans . Wild type strain used was the C. elegans isolate from Bristol (N2) [37] ; arIs37[ p myo-3::ssGFP] [38] was used for co-localization of I TMR and green fluorescent protein (GFP). Microinjections were performed as previously described [39] . Samples were injected in the dorsal side of pseudocoelom, opposite the vulva, of 1-day-old hermaphrodites. Injected worms were transferred to nematode growth medium (NGM) plates (+OP50), incubated at 22 °C for the stated time-points, and imaged. Co-localization of GFP and TMR was performed by injecting 3 μM of I TMR into arIs37 worms. Uptake assays were performed by injecting 3 μM of I FD10 alone, and with ten equivalents of mBSA, into N2 worms. The same was done with an equivalent amount of free FD10 and ten equivalents of mBSA. Injected worms were incubated for 3 h. In vivo pH measurements For the in vitro calibration curve, 150 nM of I FD10 , dissolved in 20 mM pH clamping buffer of a given pH (120 mM KCl, 5 mM NaCl, 1 mM CaCl 2 , 1 mM MgCl 2 , 20 mM HEPES), was excited at 480 nm (±10 nm) and 430 nm (±15 nm) and emission measured at 535 nm (±15 nm). The fluorescent ratios obtained were plotted against pH values to obtain a calibration curve. For the in vivo pH calibration in coelomocytes, hermaphrodites were injected with 3 μM of I FD10 and incubated for 3 h. After piercing the cuticle with a microinjection needle, the worms were immersed in pH clamping buffer of desired pH containing 100 μM of nigericin for 75 min. Coelomocytes were imaged after mounting the worms on a 2% agarose pad using clamping buffer. For real-time pH measurements, 10 hermaphrodites were injected, incubated at 22°C and, after the requisite time, incubated on ice. This cold treatment efficiently stops endocytosis. Worms were then anaesthetized using 40 mM sodium azide in M9 buffer and imaged. Image acquisition and quantification In cellulo and in vivo imaging used TE2000U microscope (Nikon), equipped with mercury arc illuminator (Nikon), Photometrics Cascade II CCD camera and Chroma dichroic and band pass filters (Chroma). Images in each experiment were acquired under the same settings, using Metamorph software (Universal Imaging). In vivo co-localization imaging was performed on Fluoview 1,000 confocal microscope (Olympus) equipped with argon ion laser for 488 nm excitation and He–Ne laser for 543 excitation with dichroics, excitation and emission filters suitable for each fluorophore. Image quantification was done using ImageJ ver. 1.42 software (NIH). Briefly, hemocyte images were background subtracted, cell boundary was determined from the bright field image and total cell intensity calculated. The mean intensity in five fields of view was obtained and normalized with respect to I FD10 alone. For the in vivo uptake assays, the number of coelomocytes labelled were counted and expressed as a percentage of the total number of coelomocytes. For in vivo pH measurements, dual excitation of I FD10 was performed. After background subtraction, endosomes were demarcated in each image and their mean intensity calculated. The ratio of mean intensities at 520 nm when excited at 480 nm as well as 430 nm gives the 480:430 ratio of each endosome. How to cite this article: Bhatia, D. et al . A synthetic icosahedral DNA-based host–cargo complex for functional in vivo imaging. Nat. Commun. 2:339 doi: 10.1038/ncomms1337 (2011).